A two-locus interaction causes interspecific hybrid weakness in rice Reproductive barriers perform a vital role during speciation. Hybrid weakness, the poorer development of hybrids compared with their parents, hinders gene exchange between different species at the postzygotic stage. Here we show that two incompatible dominant loci ( Hwi1 and Hwi2 ) involving three genes are likely to determine the high temperature-dependent expression of hybrid weakness in interspecific hybrids of rice. Hwi1 comprises two leucine-rich repeat receptor-like kinase (LRR–RLK) genes, 25L1 and 25L2 , which are specific to wild rice ( Oryza rufipogon ) and induce hybrid weakness. Hwi2, a rare allele that is predominantly distributed in indica rice ( Oryza sativa ), encodes a secreted putative subtilisin-like protease. Functional analysis indicated that pyramiding of Hwi1 and Hwi2 activates the autoimmune response in the basal nodes of hybrids, interrupting root formation and then impairing shoot growth. These findings bring new insights into our understanding of reproductive isolation and may benefit rice breeding. How species become species is one of the most fascinating enigmas in nature. Reproductive isolation, which may be caused by genetic incompatibility after fertilization, is considered to play a vital role in this process [1] . The Dobzhansky–Muller (DM) model postulates that deleterious interactions between different alleles arising from evolutionarily divergent populations result in genetic incompatibility [2] , [3] . However, our understanding of the underlying molecular mechanisms of speciation is limited. Several speciation genes, which contribute to the barriers of gene flow, have been identified in animals and plants [4] , [5] , [6] , [7] . Nevertheless, most of these studies have focused on hybrid sterility while overlooking other types of hybrid incompatibility, such as hybrid weakness, a common phenomenon referring to the retarded growth and development of hybrids in comparison to their parents [8] . Several hybrid weakness cases have been reported in crops, either at the interspecific or intraspecific level [9] , [10] , [11] , [12] , [13] , [14] , potentially hindering the full utilization of heterosis. Therefore, elucidating the molecular basis of hybrid weakness will contribute to our understanding of the science of evolution and will enhance crop breeding. Owing to its biological and evolutionary significance, hybrid weakness has gradually been attracting attention, and a few hybrid weakness genes have recently been cloned in dicots [15] , [16] , [17] , [18] , [19] , [20] . However, no causal gene for hybrid weakness has been isolated in monocots to date. Here we report that the wild rice Hwi1 locus comprises two indispensable LRR–RLK genes and genetically interacts with a subtilisin-like protease gene Hwi2 from Teqing to induce the expression of hybrid weakness by constitutively activating the autoimmunity, possibly through the ligand-receptor signalling transduction. Hybrid weakness syndrome in rice Previously, we discovered a novel type of interspecific hybrid weakness syndrome in rice [21] through analysis of a chromosome segment substitution line (CSSL) library derived from a cross between the indica variety Teqing ( Oryza sativa ) and a common wild rice ( Oryza rufipogon ) strain obtained from Hainan province, China [22] . This weakness syndrome, which is manifested by short stature and impaired root formation ( Fig. 1a,b ), is induced by the introgression of the dominant gene Hwi1 from wild rice into the Teqing background [21] . Along with the expression of weakness, we noticed that some necrotic lesions arise from basal nodes and lower parts of leaf sheaths in NIL( Hwi1 ), a nearly isogenic line (NIL) that carries the Hwi1 gene in the Teqing background ( Fig. 1b ; Supplementary Fig. 1a,b ). Examination of cross-sections of these plants revealed that the necrotic lesions are possibly caused by regional browning and shrunken parenchymal cells in basal nodes and leaf sheath ( Fig. 1c ; Supplementary Fig. 1c ). The necrotic leaf sheaths contain less chlorophyll and accumulate more lignin ( Supplementary Fig. 1d,e ). Additionally, numerous unidentified, dark compounds were observed in the vacuoles of abnormal cells ( Supplementary Fig. 1f ). These results suggest that cell death may be activated in NIL( Hwi1 ). A TUNEL assay further confirmed that the programmed cell death (PCD) status is highly increased in NIL( Hwi1 ) basal nodes compared with those of NIL( hwi1 ) ( Fig. 1d ). In general, these symptoms are similar to the characteristics of pathogen-infected plants. 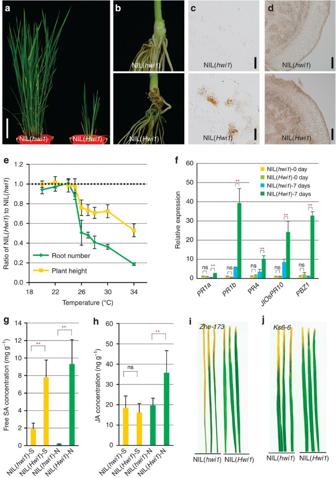Figure 1: Phenotypic and molecular characterization of rice hybrid weakness. (a) Morphology of NIL(hwi1) and NIL(Hwi1) at the booting stage. (b) Phenotype of the basal nodes of 30-day-old NIL(hwi1) and NIL(Hwi1) plants. (c) Cross-sections of the basal nodes of NIL(hwi1) and NIL(Hwi1) plants without staining; scale bar, 200 μm. (d) TUNEL assay to detect PCD status of basal nodes from 8-day-old NIL(hwi1) and NIL(Hwi1) seedlings; scale bar, 100 μm. (e) Effect of temperature treatments on the expression of hybrid weakness. (f) The expression of variousPRsin the basal nodes of NIL(hwi1) and NIL(Hwi1) plants at 0 and 7 days after shifting from 20 to 30 °C. (g) The free salicylic acid content in leaf sheaths and basal nodes of NIL(hwi1) and NIL(Hwi1). (h) The jasmonic acid content in leaf sheaths and basal nodes of NIL(hwi1) and NIL(Hwi1). (i) The resistance of NIL(hwi1) and NIL(Hwi1) to bacterial pathogenXoostrainZhe-173at the seedling stage. (j) The resistance of NIL(hwi1) and NIL(Hwi1) to bacterial pathogenXoostrainKs6-6at the seedling stage. Error bars in (e–h) indicate s.d.,n=10 (e),n=3 (f–h). **significant difference determined by thet-test atP<0.01; ns, not significant. S and N in (g) and (h) indicate leaf sheaths and basal nodes, respectively. Figure 1: Phenotypic and molecular characterization of rice hybrid weakness. ( a ) Morphology of NIL( hwi1 ) and NIL( Hwi1 ) at the booting stage. ( b ) Phenotype of the basal nodes of 30-day-old NIL( hwi1 ) and NIL( Hwi1 ) plants. ( c ) Cross-sections of the basal nodes of NIL( hwi1 ) and NIL( Hwi1 ) plants without staining; scale bar, 200 μm. ( d ) TUNEL assay to detect PCD status of basal nodes from 8-day-old NIL( hwi1 ) and NIL( Hwi1 ) seedlings; scale bar, 100 μm. ( e ) Effect of temperature treatments on the expression of hybrid weakness. ( f ) The expression of various PRs in the basal nodes of NIL( hwi1 ) and NIL( Hwi1 ) plants at 0 and 7 days after shifting from 20 to 30 °C. ( g ) The free salicylic acid content in leaf sheaths and basal nodes of NIL( hwi1 ) and NIL( Hwi1 ). ( h ) The jasmonic acid content in leaf sheaths and basal nodes of NIL( hwi1 ) and NIL( Hwi1 ). ( i ) The resistance of NIL( hwi1 ) and NIL( Hwi1 ) to bacterial pathogen Xoo strain Zhe-173 at the seedling stage. ( j ) The resistance of NIL( hwi1 ) and NIL( Hwi1 ) to bacterial pathogen Xoo strain Ks6-6 at the seedling stage. Error bars in ( e – h ) indicate s.d., n =10 ( e ), n =3 ( f – h ). **significant difference determined by the t -test at P <0.01; ns, not significant. S and N in ( g ) and ( h ) indicate leaf sheaths and basal nodes, respectively. Full size image Temperature affects the expression of hybrid weakness Interestingly, we found that the expression of hybrid weakness is temperature-dependent. Weakness syndrome did not appear at temperatures <26 °C, and the symptoms become more severe at higher temperatures ( Fig. 1e ; Supplementary Fig. 2 ; Supplementary Fig. 3a–d ). Even in plants already exhibiting hybrid weakness, symptoms could be reversed by low-temperature treatment ( Supplementary Fig. 3b,d ). Moreover, simply treating the underground parts (including the roots and the basal nodes) of the plants with high temperatures seemed sufficient to induce weakness syndrome, while the same treatment applied to above-ground parts had a very limited effect ( Supplementary Fig. 3e,f ), indicating that NIL( Hwi1 ) senses temperature in its underground parts to induce weakness syndrome. Autoimmune activation of the hybrid weakness plants We conducted microarray analysis to unravel the global changes in gene expression in 20 °C-grown seedlings after they were shifted to 30 °C conditions at day 0, 3, 7 or 15. A total of 5,852 genes in NIL ( Hwi1 ) basal nodes showed twofold or more differential expression during at least one of the four time points. K-means analysis classified these genes into six clusters ( Supplementary Fig. 4 ). We compared the gene expression patterns of each cluster with those of the corresponding genes in NIL( hwi1 ). Cluster 0 and cluster 3 exhibited dramatic alterations in expression; most genes were strikingly upregulated in NIL( Hwi1 ) but not in NIL( hwi1 ) ( Supplementary Fig. 4 ). We performed gene ontology (GO) annotation of NIL( Hwi1 )-specific differentially expressed genes from cluster 0 and cluster 3. Corresponding to the phenotypic characteristics that we observed, PCD-related and biotic stress-responding genes were highly enriched ( Supplementary Table 1 ). Some pathogen-related genes ( PRs ), including PR1a , PR1b , PR4 , JIOsPR10 and PBZ1 , did not exhibit differential expression between NIL( Hwi1 ) and NIL( hwi1 ) at 20 °C, while their expression was dramatically induced in NIL( Hwi1 ) after 7 days of 30 °C treatment ( Fig. 1f ). This findings were consistent with our previously results [21] . Furthermore, the activation of some PRs , such as PBZ1 , was always associated with the occurrence of weakness syndrome under various conditions ( Supplementary Fig. 5 ). Additionally, salicylic acid (SA) and jasmonic acid (JA), two well-known phytohormones involved in defence responses, were highly accumulated in NIL( Hwi1 ) basal nodes ( Fig. 1g,h ). The NIL( Hwi1 ) grown in sterile condition showed similar symptoms of that grown in regular condition ( Supplementary Fig. 6 ). Taken together, these results suggest that the expression of hybrid weakness may be associated with the activation of autoimmunity, which is independent of the extrinsic pathogens infection. Consistent with this notion, NIL( Hwi1 ) exhibited enhanced resistance to different strains of the bacterial pathogen Xanthomonas oryzae pv oryzae ( Xoo ) at various developmental stages ( Fig. 1i,j ; Supplementary Fig. 7 ). Gene isolation of Hwi1 and Hwi2 We previously delimited Hwi1 into a 13.2-kb region on chromosome 11, which harbours two leucine-rich repeat receptor-like kinase (LRR–RLK) genes ( LOC_Os11g07230 and LOC_Os11g07240 ), according to genomic annotation of Nipponbare ( Oryza sativa ) ( Fig. 2a ) [21] . However, complementation tests failed when we introduced wild rice genomic sequences of these two LRR–RLK genes into Teqing. Therefore, we constructed a wild rice BAC clone library and sequenced the candidate region to explore whether structural variations (SVs) exist in wild rice. Two additional LRR–RLK genes, designated as LOC_Os11g07225-like 1 ( 25L1 ) and 25L2 due to their similarity to the flanking gene LOC_Os11g07225 ( Supplementary Fig. 8 ), as well as two retrotransposon pseudogenes, were discovered in the wild rice genome ( Fig. 2b ). We transformed four overlapping genomic segments derived from a BAC clone, namely 2F2, 1H4, 1D2 and 1A3 ( Fig. 2c , which carry intact LOC_Os11g07225 and 25L1 ; 25L1 and retrotransposon pseudogenes, 25L1 , 25L2 and retrotransposon pseudogenes, and 25L2 , LOC_Os11g07230 and LOC_Os11g07240 , respectively) into Teqing for complementation testing. The segment 1D2, but not 2F2, 1H4 or 1A3, was able to induce weakness syndrome in Teqing ( Fig. 2d ; Supplementary Fig. 9a–c ), indicating that 25L1 and 25L2 are indispensable for the expression of hybrid weakness, whereas 25L1 or 25L2 alone is not sufficient for triggering its expression. Furthermore, the expression of PRs in transformants carrying the 1D2 segment was highly activated compared with that in Teqing, but this was not the case in transformants harbouring 1A3, 1H4 or 2F2 ( Fig. 2e , Supplementary Fig. 10a–c ). 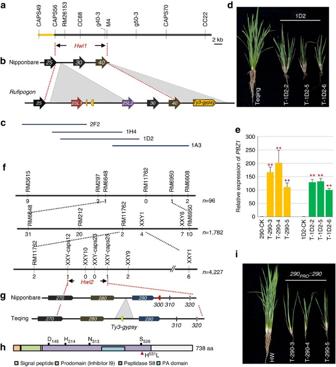Figure 2: Map-based cloning and genetic complementation ofHwi1andHwi2. (a) Gene location ofHwi1. (b) Diagram of SVs within the candidate region between Nipponbare (Oryza sativa) and wild rice (Oryza rufipogon). Arrows indicate the candidate genes. The last two digits ofLOC_Os072XXgene identifiers are given for each gene. Insertions in wild rice are indicated with grey triangles. Transposable elements or their remains are indicated with yellow pentagons. (c) Segments derived from a Hainan wild rice BAC clone used for complementation tests. (d) Independent transformants carrying 1D2 fragment in Teqing express weakness syndrome. (e) The expression levels ofPBZ1in different transgenic lines. Yellow and green colours indicate290PRO::290and 1D2 transformants, respectively. **indicates significant difference between the transgenic plants and the corresponding control determined by thet-test atP<0.01. Error bars indicate s.d.,n=3. (f) Fine mapping ofHwi2. Black bars and vertical lines indicate the chromosome and polymorphic markers, respectively. Individual numbers for mapping are listed to the right of the chromosome diagram. Numbers under markers indicate the recombinants identified between the marker andHwi2. (g) Schematic diagram ofHwi2candidate region in Nipponbare and Teqing. Genes are indicated with pentagons. The last three digits ofLOC_01g58XXXgene identifiers are given for each gene. Insert is indicated with a grey triangle. (h) Protein structure ofLOC_Os01g58290encoded subtilisin-like protease. D145, H214, N313and S526are conserved amino-acid residues of the catalytic triads. Red triangle indicates the functional mutation H531L. (i) Independent transformants with TeqingHwi2in the HW line induced the expression of hybrid weakness. Figure 2: Map-based cloning and genetic complementation of Hwi1 and Hwi2 . ( a ) Gene location of Hwi1 . ( b ) Diagram of SVs within the candidate region between Nipponbare ( Oryza sativa ) and wild rice ( Oryza rufipogon ). Arrows indicate the candidate genes. The last two digits of LOC_Os072XX gene identifiers are given for each gene. Insertions in wild rice are indicated with grey triangles. Transposable elements or their remains are indicated with yellow pentagons. ( c ) Segments derived from a Hainan wild rice BAC clone used for complementation tests. ( d ) Independent transformants carrying 1D2 fragment in Teqing express weakness syndrome. ( e ) The expression levels of PBZ1 in different transgenic lines. Yellow and green colours indicate 290 PRO ::290 and 1D2 transformants, respectively. **indicates significant difference between the transgenic plants and the corresponding control determined by the t -test at P <0.01. Error bars indicate s.d., n =3. ( f ) Fine mapping of Hwi2 . Black bars and vertical lines indicate the chromosome and polymorphic markers, respectively. Individual numbers for mapping are listed to the right of the chromosome diagram. Numbers under markers indicate the recombinants identified between the marker and Hwi2 . ( g ) Schematic diagram of Hwi2 candidate region in Nipponbare and Teqing. Genes are indicated with pentagons. The last three digits of LOC_01g58XXX gene identifiers are given for each gene. Insert is indicated with a grey triangle. ( h ) Protein structure of LOC_Os01g58290 encoded subtilisin-like protease. D 145 , H 214 , N 313 and S 526 are conserved amino-acid residues of the catalytic triads. Red triangle indicates the functional mutation H 531 L. ( i ) Independent transformants with Teqing Hwi2 in the HW line induced the expression of hybrid weakness. Full size image According to the DM model, some additional gene(s) may be required for inducing weakness syndrome. To identify the underlying gene(s), we constructed an F 2 population derived from a cross between NIL( Hwi1 ) and Zhonghua 11 ( O. sativa ssp. japonica ) and discovered that another dominant gene, Hwi2 , which originated from Teqing but is not present in Zhonghua 11 or wild rice, is essential for inducing hybrid weakness ( Supplementary Fig. 11 ). Hwi2 was narrowed down to a 35.4-kb region on chromosome 1 ( Fig. 2f,g ). Within this candidate region, LOC_Os01g58290 (abbreviated ‘ 290 ’ hereafter), which encodes a subtilisin-like protein ( Fig. 2h ), was able to trigger hybrid weakness when we transformed the Teqing allele into HW, a genetic line carrying Hwi1 in a Zhonghua 11 background lacking Hwi2 ( Fig. 2i ; Supplementary Fig. 9d ). This result confirmed that 290 is the causal gene of Hwi2 . In addition, the expression of PR genes in 290- transformants was highly upregulated ( Fig. 2e ; Supplementary Fig. 10c ), providing additional evidence that the expression of hybrid weakness is associated with autoimmunity. In the coding sequence of 290 , three single nucleotide polymorphisms (SNPs) were identified between Zhonghua 11 and Teqing, two of which are synonymous mutations, while the third mutation, A 1,592 T , encodes histidine instead of leucine (H 531 L; Fig. 2h ). H 531 does not belong to the four conserved residues of catalytic triads ( Fig. 2h ). However, this residue is highly conserved in the grass subtilisin-like protease family ( Supplementary Fig. 12 ). Therefore, we inferred that A 1,592 T is a potentially functional polymorphism. Several varieties carrying 1,592 T were crossed with another CSSL, SW115 with the Hwi1Hwi1 / hwi2hwi2 genotype. Plants exhibiting weakness were observed in the F 2 populations ( Fig. 3a,b ), and the ratio of plants exhibiting weakness: normal plants was 9:7 ( Supplementary Table 2 ). However, in the F 2 populations derived from crosses between 1,592 A -carrying varieties and SW115, no weakness was observed ( Fig. 3a,c ; Supplementary Table 2 ). These results confirm that T 1,592 A is a possible functional SNP. 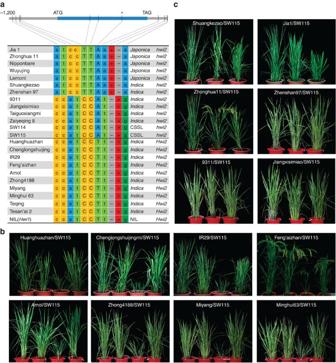Figure 3: Identification of the functional SNP ofHwi2. (a) Haplotypes ofHwi2of various germplasm. Uppercase letters indicate the SNPs in the coding sequence (shown as the blue bar), lowercase letters indicate the SNPs outside of the coding sequence (shown as the grey bars). ‘+’ and ‘−’ indicate the presence or absence of insertions, respectively. The SNP associate withHwi2/hwi2is marked with ‘*’. (b) Representative plants showed in the SW115/1,592T-carrying varieties derived F2populations. (c) Representative plants showed in the SW115/1,592A-carrying varieties derived F2populations. Plants on left and right side shown in (b) and (c) are the parents for crosses. Central plants are representative F2individuals. Figure 3: Identification of the functional SNP of Hwi2 . ( a ) Haplotypes of Hwi2 of various germplasm. Uppercase letters indicate the SNPs in the coding sequence (shown as the blue bar), lowercase letters indicate the SNPs outside of the coding sequence (shown as the grey bars). ‘+’ and ‘−’ indicate the presence or absence of insertions, respectively. The SNP associate with Hwi2/hwi2 is marked with ‘*’. ( b ) Representative plants showed in the SW115/1,592 T -carrying varieties derived F 2 populations. ( c ) Representative plants showed in the SW115/1,592 A -carrying varieties derived F 2 populations. Plants on left and right side shown in ( b ) and ( c ) are the parents for crosses. Central plants are representative F 2 individuals. Full size image We also identified four SNPs and two SNPs as well as two Indels within the 1,200 bp upstream and 500 bp downstream of the 290 -coding region, respectively ( Fig. 3a ). However, none of the variations shows association with the Hwi2 genotype. Additionally, we detected the expression level between hwi2 - and Hwi2 -carrying varieties. There was no significant expression difference between these two groups ( Supplementary Fig. 13 ), indicating the mutations locating in transcriptional regulatory sequence, such as the promoter and 5′ and 3′ UTR, may not affect the gene expression. Therefore, we targeted the polymorphic site T 1,592 A as the functional SNP. Expression pattern and subcellular localization The 25L1 , 25L2 and 290 genes were highly expressed in the basal nodes of NIL( Hwi1 ), where weakness syndrome was initially activated ( Fig. 4a–c ). Moreover, in parallel with the increased severity of the hybrid syndrome, the expression levels of these genes increased in parallel with an increase in temperature ( Fig. 4d–f ). 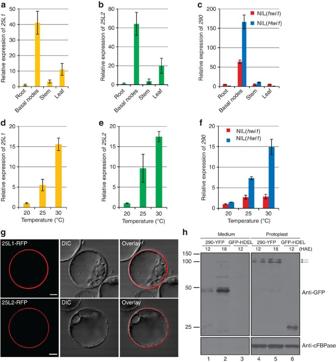Figure 4: Expression pattern of three genes and the subcellular localization of their encoded proteins. (a) Spatial expression pattern of25L1.(b) Spatial expression pattern of25L2. (c) Spatial expression pattern of and290. (d) Relative expression of25L1in the basal nodes of NIL(Hwi1) under various temperature conditions. (e) Relative expression of25L2in the basal nodes of NIL(Hwi1) under various temperature conditions. (f) Relative expression of290in the basal nodes of NIL(Hwi1) and NIL(hwi1) under various temperature conditions. (g) Transient expression of 25L1C:RFP and 25L2C:RFP fusions inArabidopsisprotoplasts for protein subcellular localization analysis. Left, middle and right panels show the fluorescence signals in cytoplasm membrane, the differential interference contrast (DIC) images and the merged images, respectively. Scale bar, 10 μm. (h) Subcellular localization analysis of 290 via immunoblot detection of 290–YFP fusion protein inArabidopsisprotoplast culture medium. Medium: fractions collected from protoplast culture medium, which represent secreted protein; Protoplast: protoplast fractions lysed via sonication, which represent intracelluar proteins; HAE, hours after electroporation; GFP-HDEL, a negative control, as this marker protein contains the C-terminal ER retention motif HDEL (His-Asp-Glu-Leu), which cannot be secreted but is instead trapped in the ER, thereby yielding no secretion band in medium fraction; cFBPase, cytosolic fructose-1,6-bisphosphatase distributed in photosynthetic tissues, used as the loading control for intracellular proteins. The upper and lower arrows indicate premature and mature 290, respectively. Molecular weight (kDa) indicated by protein markers is shown in the left. Error bars in (a–f) indicate s.d.,n=3. Figure 4: Expression pattern of three genes and the subcellular localization of their encoded proteins. ( a ) Spatial expression pattern of 25L1. ( b ) Spatial expression pattern of 25L2 . ( c ) Spatial expression pattern of and 290 . ( d ) Relative expression of 25L1 in the basal nodes of NIL( Hwi1 ) under various temperature conditions. ( e ) Relative expression of 25L2 in the basal nodes of NIL( Hwi1 ) under various temperature conditions. ( f ) Relative expression of 290 in the basal nodes of NIL( Hwi1 ) and NIL( hwi1 ) under various temperature conditions. ( g ) Transient expression of 25L1C:RFP and 25L2C:RFP fusions in Arabidopsis protoplasts for protein subcellular localization analysis. Left, middle and right panels show the fluorescence signals in cytoplasm membrane, the differential interference contrast (DIC) images and the merged images, respectively. Scale bar, 10 μm. ( h ) Subcellular localization analysis of 290 via immunoblot detection of 290–YFP fusion protein in Arabidopsis protoplast culture medium. Medium: fractions collected from protoplast culture medium, which represent secreted protein; Protoplast: protoplast fractions lysed via sonication, which represent intracelluar proteins; HAE, hours after electroporation; GFP-HDEL, a negative control, as this marker protein contains the C-terminal ER retention motif HDEL (His-Asp-Glu-Leu), which cannot be secreted but is instead trapped in the ER, thereby yielding no secretion band in medium fraction; cFBPase, cytosolic fructose-1,6-bisphosphatase distributed in photosynthetic tissues, used as the loading control for intracellular proteins. The upper and lower arrows indicate premature and mature 290, respectively. Molecular weight (kDa) indicated by protein markers is shown in the left. Error bars in ( a – f ) indicate s.d., n =3. Full size image We constructed fusions of 25L1C terminal (including the transmembrane domain and the kinase domain) and red fluorescent protein (25L1C:RFP) and 25L2C:RFP. Subcellular localization results show that 25L1 and 25L2 localize on plasma membrane ( Fig. 4g ). Notably, 290 is predicted to be a secretory protein. To verify this hypothesis, a secretion assay was performed. Proteins extracted from Arabidopsis protoplasts transformed with 290-YFP and proteins from the incubation medium were subjected to immunoblot analysis ( Fig. 4h ). For protoplastic proteins, two bands, corresponding to full-length and mature 290, were detected. For the incubation medium proteins, however, only mature 290 was detected 18 h after electroporation. Nevertheless, for some unknown reason, mature 290 appeared to be less stable in the medium than in protoplasts. These results indicate that 290 is a secretory protein. Geographic distribution of Hwi1 and Hwi2 We analysed SVs at the Hwi1 locus in the Oryza genus. Three major structures, namely Nipponbare-like (NB-like), 9311-like and Hainan wild rice-like (HN-like), which carry truncated 25L2 ( 25L2-t ), intact 25L2 * (with a different promoter from that of 25L2 ) and 25L1 and 25L2 , respectively, are widely represented ( Fig. 5a , Table 1 ). Most likely, 9311-like Hwi1 is the ancestral form, because an outgroup reference, O. glaberrima , shares the same structure with indica variety 9311. The 9311-like and NB-like Hwi1 are distributed broadly in either O. rufipogon or O. sativa , while HN-like Hwi1 seems to only be expressed in O. rufipogon ( Table 1 ). Based on whole-genome resequencing data, Huang et al . [23] classified O. rufipogon into three groups (Or-I, II and III). We found that each group contains all three SVs of Hwi1 ( Fig. 5b , Table 1 ). Even at the same or nearby geographic locations, different Hwi1 structures may coexist ( Fig. 5c ; Supplementary Table 3 ). Notably, because of the technical obstacles, we were not able to perform test-cross analysis of different wild rice strains, like what we did for Hwi2 functional SNP-carrying varieties. Therefore, if all of the HN-like strains carry Hwi1 allele need to be further confirmed. 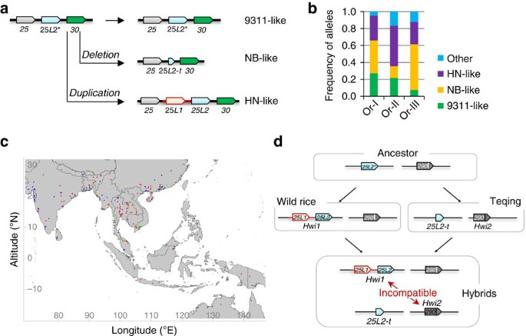Figure 5: Distribution of the allelic forms ofHwi1andHwi2and genetic model for the expression of hybrid weakness. (a) Schematic representation of different allelic forms at theHwi1locus. Red bars indicate DNA insertion.25L2*, the original allele whose promoter is different from that of25L2;25L2-t, truncated25L2, which lost the 5′-half of the gene. (b) Fraction of allelic forms ofHwi1in different subgroups of wild rice. (c) Geographical distribution of allelic forms ofHwi1in wild rice. 9311-like, NB-like, HN-like and other types ofHwi1are indicated by green, blue, red and yellow/purple, respectively. (d) Genetic model of the induction of hybrid weakness. During the evolution ofO. rufipogon, gene duplication of25L2*, which possibly caused by transposable elements, gave birth to25L1. The promoter region of25L2*was also replaced by new insertion and produced the new gene25L2.25L1and25L2compose theHwi1locus persisted in certain common wild rice strains. Forindicarice Teqing, a missense mutation event, T1,592A, was occurred athwi2locus and generated the new allele,Hwi2.Hwi1andHwi2are compatible with their own genetic background. However,Hwi1andHwi2conflict with each other in the hybrids and result in the weakness syndrome, which eventually impedes the genetic exchange. Figure 5: Distribution of the allelic forms of Hwi1 and Hwi2 and genetic model for the expression of hybrid weakness. ( a ) Schematic representation of different allelic forms at the Hwi1 locus. Red bars indicate DNA insertion. 25L2* , the original allele whose promoter is different from that of 25L2 ; 25L2-t , truncated 25L2 , which lost the 5′-half of the gene. ( b ) Fraction of allelic forms of Hwi1 in different subgroups of wild rice. ( c ) Geographical distribution of allelic forms of Hwi1 in wild rice. 9311-like, NB-like, HN-like and other types of Hwi1 are indicated by green, blue, red and yellow/purple, respectively. ( d ) Genetic model of the induction of hybrid weakness. During the evolution of O. rufipogon , gene duplication of 25L2* , which possibly caused by transposable elements, gave birth to 25L1 . The promoter region of 25L2* was also replaced by new insertion and produced the new gene 25L2 . 25L1 and 25L2 compose the Hwi1 locus persisted in certain common wild rice strains. For indica rice Teqing, a missense mutation event, T1,592A, was occurred at hwi2 locus and generated the new allele, Hwi2 . Hwi1 and Hwi2 are compatible with their own genetic background. However, Hwi1 and Hwi2 conflict with each other in the hybrids and result in the weakness syndrome, which eventually impedes the genetic exchange. Full size image Table 1 Distribution of allelic forms of Hwi1 and Hwi2 in rice. Full size table Nipponbare genomic sequence was used as the reference for resequencing short reads assembling. As the 25L1 and 25L2 are absent in Nipponbare genome, we could not obtain the SNPs information of the inserted fragment from the wild rice re-squencing data. Alternatively, we analysed the Tajima ’s D value of a wider region, which included majority part of the LRR–RLKs cluster. The Tajima ’s D value of the expanded region is 3.54 ( P <0.01), indicating the tandemly arrayed LRR–RLKs of wild rice, including 25L1 and 25L2 (owing to linkage disequilibrium), may undergo balancing selection. However, it should be noted that due to the sequence similarity, the reads from supernumerary genes may confound the estimation of the actual levels of polymorphism. Unlike Hwi1 , only 33 out of 706 cultivars and wild rice accessions carry the Hwi2 allele (1,592 T ), and almost all of these are indica varieties ( Table 1 ; Supplementary Table 4 ). Of the 340 samples that were covered by short sequencing reads at the Hwi2 locus and genotyped by PCR at the Hwi1 locus, no sample carried HN-like Hwi1 and Hwi2 (1,592 T ) simultaneously, possibly due to their deleterious interaction, which induces weakness syndrome ( Supplementary Table 5 ). The rice genome contains 309 LRR–RLKs [24] and 63 subtilisin-like proteases [25] . Duplication plays an important role in the expansion of these gene families [24] , [25] . Interestingly, Hwi1 and Hwi2 are located within tandemly arrayed LRR–RLK and subtilisin-like protease gene clusters, respectively ( Fig. 2b,g ), suggesting that gene duplication acts in reproductive isolation for species divergence. The two indispensable LRR–RLK components of Hwi1 conflict with Hwi2 to induce a hybrid weakness event ( Fig. 5d ). Identification of this two-locus/three-gene genetic system gives us a new perspective on the DM model. The number of genes involved in the regulation of genetic incompatibility may exceed that of the loci currently identified, especially for loci at tandem gene clusters. Our results show that autoimmunity is associated with the expression of hybrid weakness ( Fig. 1 ; Supplementary Figs 5,6 and 10 ), indicating that Hwi1 and Hwi2 may function in defence responses in rice. Several LRR–RLKs are employed as receptors to monitor the signalling molecules released by pathogens [26] . Endogenous signal peptides can induce immune reactions as well [27] . Recently, a subtilisin-like protein from soybean containing an embedded signal peptide was reported to activate defence-related genes [28] . In addition, several sublitisin-like proteases in plants have been identified as PR proteins [29] , [30] . Our findings show that Hwi2 is a secreted protein ( Fig. 4h ). Considering its putative serine protease activity, Hwi2 may function in protein degradation or processing out of the plasma membrane. Although the substrate of Hwi2 is unknown, it is possible that the product produced by Hwi2 acts as an internal signal to be perceived by the plasma membrane-targeted Hwi1 to activate downstream defence responses ( Fig. 6 ). Most LRR–RLKs form heterodimers in order to function [31] . Perhaps 25L1 and 25L2 interact with each other through the extracellular LRR domains to activate the ligand–receptor signal transduction pathway. 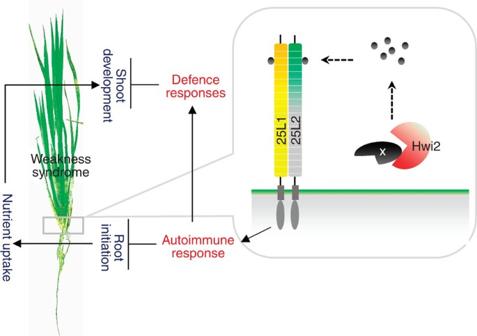Figure 6: Postulated functional model of the induction of hybrid weakness. A certain substrate X is able to be processed by Hwi2 out of the plasma membrane. The product is perceived by 25L1–25L2 membrane-targeted heterodimer to activate downstream immune responses, such as PCD and hypersensitive response-like symptoms in the basal nodes of weakness expressed plants, and impair the crown root formation. Simultaneously, the immune signal delivers to the above-ground parts. Constitutively activated defence responses suppress the growth of above-ground tissues and organs. On the other hand, the root developmental defect blocks the nutrient uptake of plant, which further impairs the growth and development. Figure 6: Postulated functional model of the induction of hybrid weakness. A certain substrate X is able to be processed by Hwi2 out of the plasma membrane. The product is perceived by 25L1–25L2 membrane-targeted heterodimer to activate downstream immune responses, such as PCD and hypersensitive response-like symptoms in the basal nodes of weakness expressed plants, and impair the crown root formation. Simultaneously, the immune signal delivers to the above-ground parts. Constitutively activated defence responses suppress the growth of above-ground tissues and organs. On the other hand, the root developmental defect blocks the nutrient uptake of plant, which further impairs the growth and development. Full size image Several examples showed that the expression of hybrid weakness is sensitive to the temperature. To our knowledge, most of the reported temperature-dependent cases, if not all, are induced by low temperature [14] , [15] , [16] , [18] , [32] . Here we reported an example of high temperature-induced hybrid weakness. As shown in the prediction model, Hwi1, comprising two indispensable cell-surface LRR–RLKs, perceive the internal signal molecule to mount pattern-triggered immunity ( Fig. 6 ). Cheng et al . [33] found that plants preferentially activate effector-triggered immunity signalling at relatively low temperatures, whereas they switch to pattern-triggered immunity signalling at moderately elevated temperatures. This discovery implies that the expression of hybrid weakness that depends on low or high temperature may be determined by the function of the causal genes. For example, Dangerous Mix 1 ( DM1 ) and DM2 -controlled hybrid necrosis of Arabidopsis is low temperature-dependent due to the underlying NB-LRR genes [15] , which may function in effector-triggered immunity pathway. It is well known that high temperature may decrease the resistance of plants [34] . However, a few examples of high temperature-activated resistance, such as Xa7 -mediated rice bacteria blight resistance [35] and Yr36 -mediated wheat strip rust resistance [36] , were discovered. Therefore, another possibility for our case is that Hwi1 and Hwi2 function in high temperature-triggered resistance of rice to induce the hybrid weakness event. Underground high-temperature treatment is sufficient to trigger weakness syndrome in roots as well as shoots ( Supplementary Fig. 3e,f ), suggesting that the thermosensor that functions in the temperature-sensitive hybrid weakness event is situated in underground tissues. Furthermore, since 25L1 , 25L2 and Hwi2 are dominantly expressed in the basal nodes ( Fig. 4a–c ), which display a much more severe phenotype than roots, perhaps the basal nodes monitor fluctuations in temperature. In according with this, we found the activation of PRs in the basal nodes was more prominent than that in the roots ( Supplementary Fig. 6e–g ). Taken together, the basal nodes may be the place where the hybrid weakness initially expressed. Highly accumulated SA in the leaf sheathes ( Fig. 1g ) and strikingly increased resistance to bacteria pathogen Xoo in leaves were observed in the plants exhibiting weakness ( Fig. 1i,j ), suggesting that the activated defence responses can be relayed from the basal nodes to the above-ground parts, which eventually hinder the shoot growth ( Fig. 6 ). This is supported by our previously findings that exogenous SA treatment was able to suppress NIL( hwi1 ) and NIL( Hwi1 ) shoot growth and made the plant height comparable [21] . On the other hand, as root development is impaired in weakness plants [21] , nutrient uptake defects may also enhance the growth suppression of the above-ground parts. These findings broaden our knowledge of the underlying mechanisms of reproductive isolation in evolution and have practical significance for plant breeding to maximally utilize invaluable genes from wild germplasm. Plant material and growth conditions The CSSL library was derived from a cross between Teqing as the recurrent parent and a common wild rice strain obtained from Hainan province, China, as the donor parent [22] . CSSL 05-SW52, which exhibited weakness syndrome, was backcrossed with Teqing and the derived segregating population was used for Hwi1 mapping. NIL( Hwi1 ) and NIL( hwi1 ), possessing an almost consistent genetic background except for a small region around the Hwi1 locus ( Supplementary Fig. 1a ), were developed from the BC 4 F 2 generation, and the genotypes were verified using whole genome-covering markers. NIL( Hwi1 ) was crossed with some japonica varieties, including Zhonghua11, Nipponbare and Wuyujing, to construct populations for Hwi2 detection and mapping. CSSL SW115, which carries substituted segments from wild rice both at the Hwi1 and Hwi2 loci, was utilized to confirm the mapping results and to test the distribution of Hwi2 in different cultivars. A HW line carrying Hwi1 but without Hwi2 was derived from a cross between Zhonghua 11 and NIL( Hwi1 ) and used for the complementation test of Hwi2 . Plants for temperature-related experiments, root number and plant height quantification and histological analysis were incubated in Yoshida’s culture solution in a growth chamber. The plants were grown under a 10 h dark/14 h light cycle at 50% humidity. For the temperature-shift experiment, plants were grown at 20 °C or 30 °C from germination to 7 weeks and then shifted to 30 °C or 20 °C. A thermostat water bath was used to control the underground temperature and air conditioning was used to control the above-ground temperature for independent above-/underground temperature assays. Mapping of Hwi2 The rough location of Hwi2 was detected by quantitative trait loci (QTL) mapping using a NIL( Hwi1 )/Zhonghua 11 F 2 population comprising 96 plants. Sixty-five SSR markers that nearly evenly covered the whole genome of rice were utilized ( Supplementary Data 1 ). QTL mapping results were analysed via R/qtl [37] , an add-on package for the command-line-based open-source statistical software programme R ( www.R-project.org/ ). By regarding hybrid weakness as a binary trait and conferring normal and weakness phenotypes a value of ‘1’ and ‘2’, respectively, both one-QTL and two-QTL models were applied to calculate the QTLs controlling hybrid weakness. Individuals carrying homozygotic Hwi1 and heterozygotic Hwi2 were selected from NIL( Hwi1 )/ japonica -derived populations, and their offspring were utilized for Hwi2 fine mapping. Indel markers for fine mapping were developed by comparing the sequences of Nipponbare and 9311. Cleaved Amplified Polymorphic Sequence (CAPS) markers were designed through BlastDigester [38] , a free online tool for CAPS development. The phenotype of each individual was evaluated in the paddy fields at Shanghai and Sanya, Hainan province, China. The seeds of recombinants were gathered and grown in the next planting season for progeny testing. Phenotypic characterization and histological analysis The number of roots of NIL( Hwi1 ) and NIL( hwi1 ) was counted and their plant heights were measured every 7 days for the time-course experiments under low (20 °C) or high (30 °C) temperature conditions. The plant heights of the seedlings were measured as the distance from the basal nodes to the uppermost tips of the leaf blades. Plant materials for histological analysis were fixed in FAA (50% ethanol, 5% glacial acetic acid and 5% formaldehyde) overnight. The samples were then embedded in Epon812 resin (Fluka) and polymerized at 60 °C. Three-micrometre-thick sections were cut and stained with filtered 1% toluidine. Sixteen-nanometre-thick sections were cut in series with an ultramicrotome (Leica EM UC6) and stained with uranyl acetate and lead citrate for transmission electron microscopy analysis. The sections were examined with a Hitachi H7650 electron microscope at 80 kV. Chlorophyll and lignin determination Chlorophyll was measured using a spectrophotometric method [39] . Leaf sheaths of NIL( Hwi1 ) and NIL( hwi1 ) were cut into small pieces and weighed, then treated with 20 ml of 80% acetone for 24 h in the dark and shaken every few hours. The clear extract was transferred to a 1.0 cm cuvette and the absorbance was measured at 645 and 663 nm. The chlorophyll a concentration was calculated using the following equations: (12.7 × OD 663 −2.59 × OD 645 ) × extraction volume/fresh weight (g); chlorophyll b concentration equals (22.9 × OD 663 −4.67*OD 645 ) × extraction volume/fresh weight (g). For lignin measurement, the cell walls were isolated as described by Turner and Somerville [40] . For each sample, the leaf sheaths of three individuals were collected, homogenized in liquid nitrogen and ground to a fine powder with a mortar and pestle. The crude cell wall fraction was obtained by extracting the soluble material three times with 70% ethanol at 70 °C for 1 h each time. The ethanol was removed from the samples and dried at 50 °C to constant weight. Lignin contents were determined following the procedure of Musel et al . [41] The cell wall materials were treated with 0.3 ml thioglycolic acid and 1.5 ml 2 mol l −1 HCl in a 2 ml tube at 95 °C for 4 h. The samples were cooled to room temperature and centrifuged (15,000 g ) for 15 min to collect the pellets. After three washes with distilled water, the pellets were treated with 1.5 ml 0.5 mol l −1 NaOH for 16 h (20 °C with shaking) to extract the lignothioglycolic acid (LTGA). The supernatant obtained after centrifugation (15,000 g , 15 min) and a second supernatant obtained after re-extracting the pellet with 0.4 ml NaOH were combined and acidified with 0.3 ml concentrated HC1. The samples were mixed and incubated for 4 h at 4 °C to precipitate the LTGA. The LTGA was recovered by centrifugation (15,000 g , 20 min) and dissolved in 1 ml 0.5 mol 1 −1 NaOH. The absorbance was measured against a NaOH blank at 280 nm, and OD 280 mg −1 of cell wall material was used to determine the relative content of lignin. Microarray analysis Plants were cultivated at constant 20 °C for 20 days and then shifted to constant 30 °C conditions. The basal nodes of NIL( Hwi1 ) and NIL( hwi1 ) were harvested immediately before the temperature shift (set as the 0 point) or at 3, 7 or 15 days after the shift. Three biological replicates (each comprising basal nodes from 15–20 individuals) were used for each time point. Total RNA extraction, cDNA and labelled cRNA synthesis and Affymetrix expression GeneChip hybridization were conducted by Shanghai Biotechnology Corporation. Data analysis, including mining of differentially expressed genes and K-mean analysis, were conducted using the microarray analysis software Genespring GX10.0. Differentially expressed genes (exhibiting at least twofold changes in expression) were screened via one-way ANOVA ( P ≤0.05). GO enrichment analysis was conducted with agriGO ( bioinfo.cau.edu.cn/agriGO/ ) using the Singular Enrichment Analysis (SEA) method and choosing the rice Affymetrix Genome Array (GPL2025) as the reference. The Yekutieli (FDR under dependency) method was used to perform multi-test adjustment ( P ≤0.05). TUNEL assay The PCD status of the basal nodes was detected using a DeadEnd Colorimetric TUNEL system (Promega) using the manufacturer’s protocol. Paraffin-embedded sections were immersed into fresh xylene twice (5 min each) in a Coplin jar. The deparaffinized slides were washed in 100% ethanol for 5 min at room temperature. Then, the samples were rehydrated by sequentially immersing the slides through graded ethanol washes (100, 95, 85, 75 and 50%) for 3 min each. Next, the slides were washed in 0.85% NaCl and PBS for 5 min each. The tissue sections were fixed by immersing the slides in 10% buffered formalin in PBS for 15 min. After two washes in PBS for 5 min each, 100 μl 20 μg ml −1 Proteinase K solution was added to each slide to cover the tissue section, and the slides were incubated for 15 min at room temperature. The slides were washed in PBS for 5 min, and the tissue sections were refixed by immersion in 10% buffered formalin in PBS for 5 min. After two additional 5-min PBS washes, the sections were equilibrated with 100 μl equilibration buffer for 10 min. Then, 100 μl of rTdT reaction mixture (98 μl equilibration buffer, 1 μl biotinylated nucleotide mix and 1 μl rTdT enzyme) was added to each slide, and the slides were covered with plastic coverslips to evenly distribute the reagents. Then, the slides were incubated in the dark at 37 °C for 60 min. The reaction was terminated by immersing the slides in 2 × SSC for 15 min, followed by three washes (5 min each) in PBS. To block endogenous peroxides, the slides were immersed in 0.3% hydrogen peroxide in PBS for 5 min. An additional three washes in PBS were conducted, and each slide was incubated in 100 μl Streptavidin HRP solution for 30 min at room temperature. After washing three times in PBS, DAB solution was added in each slide and removed by rinsing in deionized water until a light brown background appeared (~10 min). Finally, the slides were mounted and the staining was observed. Pathological analysis Rice plants were inoculated with Xoo strains Zhe-173 or Ks6-6 at the seedling and tillering stages using the scissor-dip method [42] . Lesion length was measured with a ruler at 2 weeks after inoculation to evaluate the resistance of the plants against pathogens. Measurement of free SA and JA levels Free SA and JA were extracted from 100 mg basal nodes and blade sheathes of NIL( Hwi1 ) and NIL( hwi1 ) (harvested from 15–20 plants grown at 30 °C for 30 days) and quantified via LC-MS as described previously [43] . The tissues were frozen in liquid N 2 immediately and ground to a fine powder. Homogenates were extracted in extraction buffer (1.0 ml of 80% methanol) at 4 °C overnight. The samples were centrifuged at 15,200 g for 10 min. The residues were re-extracted with 1.0 ml of 80% methanol. The combined supernatants were vacuum-dried at –60 °C, dissolved in 200 μl of 0.1 M sodium phosphate buffer (pH 7.8) and extracted with 400 μl of petroleum ether. A Sep-Pak C18 cartridge (Waters, Milford, MA, USA) was used for aqueous phase purification. The cartridge was washed with 800 μl of ddH 2 O or 1.5 ml of 50% methanol to collect the SA and JA, respectively. The eluate was vacuum-dried and dissolved in 50 μl of 20% acetonitrile for the LC/MS assay. A 5-μl aliquot of the sample was injected onto an Acquity UPLC BEH C18 column (2.1 × 100 mm, 1.7 μm, Waters, Milford, MA, USA) at 30 °C. The mobile phase, comprising solvent A (10% aqueous acetonitrile) and solvent B (acetonitrile), was used in a gradient mode. The eluant flow rate was 0.25 ml min −1 . The mass spectrometer was set to collect data in the selected ion recording mode using electrospray ionization (ESI) in the negative ion mode. The optimized conditions were as follows: capillary voltage 2.8 kV, source temperature 120 °C, desolation temperature 350 °C, desolation gas flow 600 l h −1 , cone gas flow 50 l h −1 and molecular ion m / z 137 and 209.2 for SA and JA, respectively. DNA and RNA isolation and quantitative real-time PCR Micro-quantities of rice DNA were isolated from fresh leaves as described by Lin et al . [44] Total RNA was isolated from different rice tissues grown at different temperature conditions using TRIzol reagent (Invitrogen). A PrimerScript RT Reagent Kit (TaKaRa) was utilized to synthesize cDNA according to the manufacturer’s instructions. Quantitative real-time PCR was performed in an ABI-7300 platform with SYBR Premix Ex Taq II (Perfect Real Time; TaKaRa). The reaction conditions were 95 °C for 30 s, 95 °C for 5 s and 60 °C for 31 s for 40 cycles. The actin gene was utilized as the endogenous control for normalization. The ΔΔ C t method was used for data analysis. Each real-time PCR analysis was performed using three biological replicates. The sequences of the primers used for real-time PCR are listed in Supplementary Table 6 . Analysis of Hwi1 and Hwi2 distribution Three primer sets ( Supplementary Table 6 ) were designed to determine the Hwi1 locus genotypes of 414 wild rice accessions collected worldwide. The functional SNPs at the 1,592nd position of Hwi2 CDS were used to determine the genotype. If the accession carried 1,592 T , it was thought to carry Hwi2 , while if the accession carried 1,592 A , it was regarded as carrying hwi2 . SNP information from >1,500 rice accessions was obtained from RiceHap3 ( www.ncgr.ac.cn/RiceHap3 ). Owing to the low coverage for the resequencing data, 706 accessions having short reads covering this functional SNP were identified. BAC clone library construction and sequencing A Hainan wild rice BAC clone library was constructed by Bio S&T Inc. Hainan wild rice genomic DNA isolated from etiolated leaves was partially digested with HindIII and inserted into the BAC construction vector plndigoBAC-5. The average insert size in the BAC library was 107 kb. A Teqing BAC library was ordered from the Arizona Genomics Institute ( www.genome.arizona.edu/fpc/rice/ ). The BAC clones were cultured with LB medium. PCR was employed to screen for BAC clones carrying the Hwi1 and Hwi2 candidate genes using liquid BAC clone cultures as templates and fine-mapping primers for the reactions. Positive BAC clones were verified by end sequencing. Fragments from clones with the proper insert size were subcloned and sequenced using an ABI 3730 system. Complementation test To construct the Hwi2 complementation vector, a Teqing BAC clone harbouring the 290 gene was used as the template to amplify genomic DNA. Since the 9.13 kb segment was too large, the entire DNA fragment was obtained by ligating two overlapping short fragments, 290C1 and 290C2, which were amplified by high-fidelity polymerase KOD (Takara) and loaded into transition vector pTA2. Then, the Sph 1- and EcoR I-digested 9.13-kb fragment was attached to the binary vector pCAMBIA1301 using T4 ligase. A sequence-confirmed recombinant was then transformed into Agrobacterium tumefaciens strain EHA105 by electroporation (2.0 kV, 200 Ω, 25 μF) and used for plant transformation as described previously. To create the complementation constructs for Hwi1 , a 100-kb wild rice BAC clone harbouring the Hwi1 candidate region was partially digested with Sau 3AI. The 20–40 kb digested fragments were recovered and ligated to BamHI-digested binary vector pYLTAC747-SacB [45] with T4 ligase. Then, the vectors with insertions were transformed into E . coli strain DH10B by electroporation (2.0 kV, 200 Ω, 25 μF). The subclones were screened by PCR to roughly identify the inserted fragments. Four overlapping constructs, 2F2, 1D2, 1A3 and 1H4, which harboured different genes within the candidate regions, were subjected to end-sequencing to precisely identify the inserted fragments. The verified subclones were used for plant transformation. Subcellular localization Fragments 25L1C and 25L2C , which contained the transmembrane domains and the kinase domains of 25L1 and 25L2 , were amplified from NIL( Hwi1 ) cDNA using high-fidelity polymerase KOD (Takara). The full-coding sequence of Hwi2 was amplified from Teqing. The 25L1C and 25L2C , and Hwi2 fragments were digested with SpeI and XhoI and inserted into pBI221 vectors containing signal peptide and RFP, and YFP, respectively, and used for subcellular localization. The 25L1C:RFP and 25L2C:RFP constructs were transiently expressed in Arabidopsis protoplasts produced from suspension culture cells as described by Miao and Jiang [46] . The subcellular localization of these proteins was evaluated using a confocal laser scanning microscope (FluoView FV1000; Olympus). For Hwi2 subcellular localization analysis, medium fractions were collected from protoplast culture medium for secreted proteins isolation. Anti-cFBPase (Agrisera) were applied as a loading control for intracelluar protein [47] and anti-rabbit IgG-HRP (Bio-Rad) were used as secondary antibody for signal detection. GFP-HDEL was used as a negative control owing to this marker protein contains the C-terminal ER retention motif HDEL (His-Asp-Glu-Leu), GFP-HDEL cannot be secreted but be trapped in the ER, thereby yielding no secretion band in medium fraction [48] . Evaluation of Tajima’s D The genotypes of the tandemly arrayed LRR–RLK cluster (chr11: 3,570,000–3,651,500 bp, which is in corresponding to the region from LOC_Os11g07060 to LOC_Os11g07270 ) of 466 wild rice accessions were obtained from RiceHap3 www.ncgr.ac.cn/RiceHap3 . Tajima D statistic was calculated using DnaSP software version 4.0 (ref. 49 ). Accession codes: The 25L1 , 25L2 and 290 genes sequences have been deposited in GenBank nucleotide database under the accession codes KJ410135 , KJ410136 and KJ410137 , respectively. The microarray data have been deposited in Gene Expression Omnibus (GEO, http://www.ncbi.nlm.nih.gov/geo ) with GEO Series accession number GSE54243 . How to cite this article: Chen, C. et al . A two-locus interaction causes interspecific hybrid weakness in rice. Nat. Commun. 5:3357 doi: 10.1038/ncomms4357 (2014).